Diameter-dependent ion transport through the interior of isolated single-walled carbon nanotubes Nanopores that approach molecular dimensions demonstrate exotic transport behaviour and are theoretically predicted to display discontinuities in the diameter dependence of interior ion transport because of structuring of the internal fluid. No experimental study has been able to probe this diameter dependence in the 0.5–2 nm diameter regime. Here we observe a surprising fivefold enhancement of stochastic ion transport rates for single-walled carbon nanotube centered at a diameter of approximately 1.6 nm. An electrochemical transport model informed from literature simulations is used to understand the phenomenon. We also observe rates that scale with cation type as Li + >K + >Cs + >Na + and pore blocking extent as K + >Cs + >Na + >Li + potentially reflecting changes in hydration shell size. Across several ion types, the pore-blocking current and inverse dwell time are shown to scale linearly at low electric field. This work opens up new avenues in the study of transport effects at the nanoscale. Various types of nanopores and nanochannels have attracted significant interest in recent years [1] . Examples include silicon-based nanopores [2] , [3] , [4] , [5] , [6] , [7] , which achieve selectivity primarily through size-exclusion of macromolecules, and biological nanopores [8] , [9] , [10] , [11] , [12] , which manipulate their shape or present a specific pore opening to allow the passage of only specific ions such as potassium [8] , calcium [9] or sodium [9] . Single-walled carbon nanotubes (SWNTs) are promising candidates for nanopore studies [13] , [14] , [15] , [16] , [17] , [18] , [19] , [20] , [21] as they can match the well-defined diameter and high aspect ratios of traditional silicon nanopores with sub-2 nm diameters and hydrophobic interior that allows for ion selectivity. These properties potentially allow for interesting desalination [22] and DNA-sequencing applications [13] , as well as the ability to probe basic fluid structure properties at the smallest of possible scales. For this reason, a large number of molecular simulations have demonstrated interesting diameter-dependent phenomena such as ion selectivity [15] , [22] , rapid proton conduction [18] , [23] that can be caused by the unique water structures and geometric confinements [24] , [25] , [26] , and altered water-ice phase behaviour [27] . However, most studies have focused on theoretical simulations, and their experimental verification is still a subject of debate [28] , [29] , [30] , [31] . In previous work [32] , [33] , we demonstrated pore-blocking transport phenomena through the interior of multiple parallel SWNTs with lengths of approximately 1 mm. We attributed discrete stochastic changes in the measured current to the blocking of a large proton current by translocating ions based on a number of experimental observations. First, we noticed a large dependence of the blocking current on the solution pH, suggesting that protons were the majority charge carriers. Second, we only observed pore-blocking phenomena in electrolyte solutions (for example, KCl, as opposed to water, or HCl) and only with relatively small cations, suggesting that cations, not anions, were responsible for the pore-blocking phenomena. Finally, we noted that the pore-blocking phenomena are quantitatively altered with various cation species, an observation which we further explore in this work with new single-SWNT devices. In follow-up work, we were able to further demonstrate pore-blocking phenomena through multiple parallel SWNTs resulting in a stochastic three-state system [32] . Other groups have studied transport through larger collections of SWNTs [22] , [28] , [29] or with much shorter lengths [1] , [21] , but stochastic pore-blocking was not observed under these conditions. In this work, we employ a modified version of the platform introduced earlier [33] for explicit study of cation transport through single isolated SWNT that are measured and assigned a diameter and electronic type using single-molecule Raman spectroscopy. These diameter-assigned devices are used to probe the diameter dependence of pore-blocking phenomena for the first time. We then rationalize the observations using an electrochemical transport model drawing from previous literature simulations. Finally, we report the dependence of stochastic transport rates on cation type and temperature. Fabrication and characterization of single-SWNT devices Aligned SWNTs were grown on a silicon wafer by chemical vapour deposition (CVD) as in previous work [33] and characterized via Raman spectroscopy ( Fig. 1a ). The position of each SWNT was marked with e-beam evaporation ( Fig. 1b ). Raman spectra were then collected for each identified SWNT (see Methods, Supplementary Figs S1–S3 and Supplementary Table S1 ). The position of the radial breathing mode (RBM) ω RBM , a sharp peak between 100 and 300 cm −1 shown in Fig. 1c , was used to assign the SWNT diameter D SWNT via the empirical literature relation ω RBM =(248/ D SWNT ) [34] . The metal/semiconductor nature of the SWNT was determined by analysing the shape of the G peak. A strong second peak ( Fig. 1c , lower) in the G peak region indicated a metallic SWNT and the absence of such a peak ( Fig. 1c , upper) indicated a semiconductor SWNT. To prevent the use of SWNTs in a substantial narrowing that can affect the observation of the transport phenomena, we measured Raman spectra for over two or three positions along its length axis. The distance between measured points was at least 100 μm. 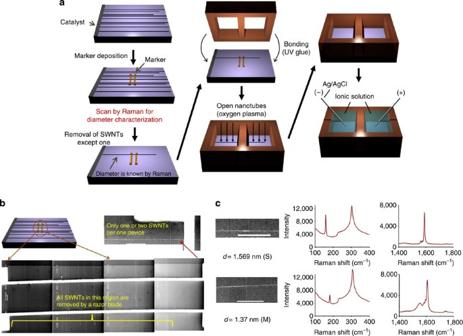Figure 1: Experimental method for manufacturing single-SWNT devices. (a) Aligned single-walled carbon nanotubes (SWNTs) are grown on a silicon wafer, identified with a marker, diameter characterized with Raman spectroscopy, all but one or a few SWNT removed with a razor blade, a two-reservoir epoxy structure bonded to the wafer, SWNT ends opened with oxygen plasma etching, and finally devices are tested with Ag/AgCl electrodes with various electrolyte solutions. (b) Example of scanning electron microscope (SEM) identification of all aligned SWNT grown on a device with the chosen SWNT for study marked. Scale bar for the SEM indicates 100 μm. (c) SEM microscope images of two representative 1.569 and 1.37 nm SWNTs (left), scale bar for the SEM indicates 100 μm. Raman characterization of the diameter of the chosen SWNT based on the radial breathing mode, and metallic/semiconductor nature based on G-peak (right). Figure 1: Experimental method for manufacturing single-SWNT devices. ( a ) Aligned single-walled carbon nanotubes (SWNTs) are grown on a silicon wafer, identified with a marker, diameter characterized with Raman spectroscopy, all but one or a few SWNT removed with a razor blade, a two-reservoir epoxy structure bonded to the wafer, SWNT ends opened with oxygen plasma etching, and finally devices are tested with Ag/AgCl electrodes with various electrolyte solutions. ( b ) Example of scanning electron microscope (SEM) identification of all aligned SWNT grown on a device with the chosen SWNT for study marked. Scale bar for the SEM indicates 100 μm. ( c ) SEM microscope images of two representative 1.569 and 1.37 nm SWNTs (left), scale bar for the SEM indicates 100 μm. Raman characterization of the diameter of the chosen SWNT based on the radial breathing mode, and metallic/semiconductor nature based on G-peak (right). Full size image After characterization of all SWNT on each wafer, one, two or three SWNTs were chosen for study, all remaining SWNTs were removed with a razor blade, and a microfluidic platform was fabricated on top as in previous work [33] ( Fig. 1a ). Briefly, the wafer was covered by an epoxy structure constructed from SU-8-negative photoresist with defined reservoirs and a 1-mm barrier region perpendicular to the SWNT alignment. The exposed ends of the SWNT were removed using oxygen plasma leaving open SWNTs that spanned the epoxy barrier. The reservoirs were then filled with electrolyte solutions and Ag/AgCl electrodes added to determine the ionic current between the reservoirs at fixed voltage differences. Electrolyte solutions were all slightly acidic from exposure of di-ionized (DI) water-based solution to air. Approximately 200 such devices were fabricated in this manner with a controlled number of SWNT and SWNT diameters spanning 0.94–2.1 nm. We observed a roughly similar successful device yield—defined as the observation of regular stochastic current fluctuations in response to the application of both an electric field and electrolyte solutions to both reservoir—of approximately 10% (see Methods, Supplementary Notes 1,2 and Supplementary Fig. S4 ). In pore-blocking events, fast proton flux [23] through the interior of SWNT results in a high current level, depleting the proton concentration in the near-pore region and increasing the concentration of cations near the pore mouth ( Fig. 2a ). Next, cations enter the SWNT and obstruct the proton flux, resulting in a low current level ( Fig. 2b ). Once the blocker emerges from the other side, the high current level is rapidly restored because of the high proton concentration near the pore mouth [33] ( Fig. 2c ). 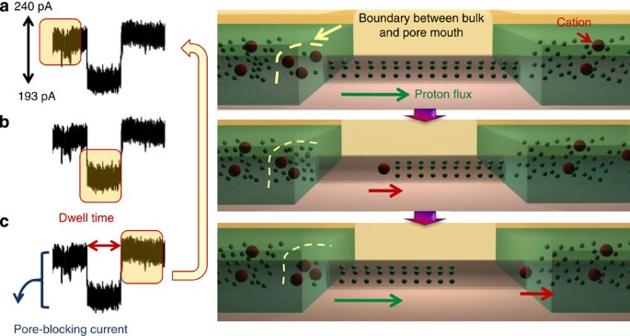Figure 2: Schematic illustration of ion transport and pore blocking in SWNTs. (a) Proton flux, (b) ion insertion (blocked by cations) and (c) recovery of proton flux. Figure 2: Schematic illustration of ion transport and pore blocking in SWNTs. ( a ) Proton flux, ( b ) ion insertion (blocked by cations) and ( c ) recovery of proton flux. Full size image Cation dependence and voltage scaling of transport phenomena We first investigated the influence of ion type and applied voltage on the observed stochastic transport phenomena using several single-SWNT devices with an unassigned diameter. 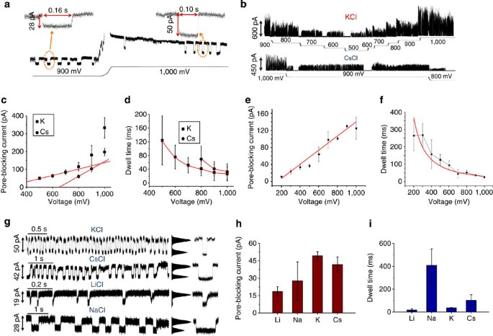Figure 3: The effect of cation type on pore-blocking phenomena. (a) Example of pore-blocking phenomena tested with 3 M KCl at two applied voltages. (b) Voltage-scanning experiment for a single SWNT with two cation types at several voltages. (c,d) Tabulated data for the effect of voltage on pore-blocking current and dwell time for potassium and cesium ions. (e,f) Effect of voltage on pore-blocking current and dwell time for a divalent cation, calcium. (g) Qualitative demonstration of the impact of four cation types on pore-blocking phenomena (left), as well as current histograms clearly demonstrating two-state oscillations. The expanded raw data (right) show distinctive pore-blocking current and dwell time behaviour as cation types are changed. (h,i) Tabulated data for the effect of cation type on observed pore-blocking current and dwell time. Figure 3a shows typical, unprocessed current traces for a voltage stepping experiment using 3 M KCl solution. At an applied voltage of 900 mV, stochastic current fluctuations are observed with a dwell time of 0.16 s and a pore-blocking current I BC of 28 pA. After increasing the applied voltage to 1,000 mV, stochastic pore blocking is re-established but with a decreased τ of 0.10 s and an increased I BC of 50 pA. This testing process was repeated for a range of voltages between 500 and 1,000 mV, and for both K + and Cs + cations through the same tube, illustrated in Fig. 3b . The average pore-blocking current and dwell time for K + and Cs + cations in another SWNT device were tabulated as a function of applied voltage for each cation and shown in Fig. 3c,d , respectively. The average pore-blocking current increased monotonically with applied voltage with a linear low-voltage regime described by our model of pore-blocking below with nonlinear, convex deflection at large voltages, whereas the dwell time decreases monotonically. From a simple scaling analysis, we expect that the pore-blocking current will scale linearly with the electric field inside the tube, calculated as the potential drop per unit length or Δ I (Δ V –Δ V t )/ L , where Δ V is the applied voltage difference across the two reservoirs, Δ V t is the threshold voltage loss across the pore observed previously [32] and the minimum voltage to observe pore-blocking phenomena, and L is the length of the connecting SWNT. Similarly, we expect that the dwell time will scale as τ = L /[(Δ V –Δ V t ) μ eff ], where μ eff is an effective ion mobility taking into account both diffusive and convective effects. These relations can also be recovered using a series expansion of the nonlinear model below to first order for small electric fields. The minimum voltage Δ V t to observe stochastic blocking is larger for cesium ions (800 mV) than for potassium ions (500 mV), consistent with an electrostatic barrier to pore transport, as observed earlier [32] . We show similar measurements for a divalent cation, Ca 2+ , in Fig. 3e,f , which shows a Δ V t of 200 mV, and follows similar scaling relationships (solid line). Also, it should be noted that lower concentration of salt (K + , Cs + , Ca 2+ ) caused the long unblocked durations and the pore-blocking events would be rare events because this condition would decrease the probability of the penetration of blockers inside of SWNTs. Figure 3: The effect of cation type on pore-blocking phenomena. ( a ) Example of pore-blocking phenomena tested with 3 M KCl at two applied voltages. ( b ) Voltage-scanning experiment for a single SWNT with two cation types at several voltages. ( c , d ) Tabulated data for the effect of voltage on pore-blocking current and dwell time for potassium and cesium ions. ( e , f ) Effect of voltage on pore-blocking current and dwell time for a divalent cation, calcium. ( g ) Qualitative demonstration of the impact of four cation types on pore-blocking phenomena (left), as well as current histograms clearly demonstrating two-state oscillations. The expanded raw data (right) show distinctive pore-blocking current and dwell time behaviour as cation types are changed. ( h , i ) Tabulated data for the effect of cation type on observed pore-blocking current and dwell time. Full size image The cation type (K + , Cs + , Li + , Na + ) was then varied for a single device with a single anion type (Cl − ) resulting in regular stochastic fluctuations with a range of dwell times and pore-blocking current, shown in Fig. 3g . Interestingly, the average pore-blocking currents and dwell time, shown in Fig. 3h,i , exhibit a non-intuitive scaling with K + >Cs + >Na + >Li + for the former and Li + <K + <Cs + <Na + for the latter. The rapid transport of Li + seems to be consistent with our previous observations [33] , despite its larger bulk ionic radius [35] . The unique scaling of these transport parameters may reflect changes in hydrated radius from bulk to a nano-confined environments, induced by shedding its hydration shells of ions to enter the molecular confined nanochannels and suggest future theoretical studies on the solvation structure of cations within SWNTs. We note that the strong dependence of blocking phenomena on cation type reinforces our understanding that the cation is central to the blocking mechanism, as we have previously observed [32] , [33] . Diameter dependence of transport phenomena Differences in stochastic pore-blocking phenomena for 12 devices with a single connecting SWNT of varying diameter reveal the first direct experimental demonstration of strongly non-monotonic diameter dependence. 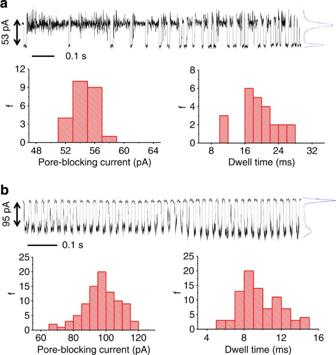Figure 4: Pore blocking for two single-SWNT devices with different SWNT diameters. (a) 1.74 nm, (b) 1.67 nm, tested at the same applied voltage (1 V) and electrolyte solution (3 M KCl). Figure 4 shows current traces and dwell time/pore-blocking current histograms for two single-SWNT devices, one with a diameter of 1.74 nm ( Fig. 4a ) and the other with a diameter of 1.67 nm ( Fig. 4b ), both using a 3 M KCl solution and applied voltage of 1,000 mV. The device with the smaller 1.67 nm diameter shows qualitatively different pore-blocking phenomena and has a much larger pore-blocking current (95 pA compared with 53 pA) and much smaller dwell time (9 ms compared with 16 ms). Despite the small difference in diameter, there is a large disparity in blockade current, contrary to a simple hypothesis that transport rates increase monotonically with diameter, as would be expected for a larger nanopore with bulk-like transport [3] , [36] . Figure 4: Pore blocking for two single-SWNT devices with different SWNT diameters. ( a ) 1.74 nm, ( b ) 1.67 nm, tested at the same applied voltage (1 V) and electrolyte solution (3 M KCl). Full size image Exploring this disparity further, the dependence of transport phenomena on SWNTs with diameters between 0.94 nm and 2.01 nm is presented in Fig. 5a , revealing that proton transport in SWNTs is at a local maximum at approximately 1.6 nm. Data collected from single-SWNT devices are shown in blue, whereas data from devices intentionally containing two or three SWNT are depicted in black, all using a 3 M KCl solution and applied voltage of 1,000 mV, and identical fabrication conditions. The scatter plot from single-SWNT devices was constructed first. From an analysis of only single-SWNT containing devices, there is a statistically significant enhancement at 1.63 nm (a Student’s t -test suggests that the maximum at 1.6 nm is statistically significant from the other devices with P <10 −6 ). We note a main peak at 1.6 nm ( Fig. 5b ), and two significant but smaller increases in pore-blocking current at the limits of the diameter range (0.94 and 2.01 nm), but no clear maximum in the dwell time ( Fig. 5c ). Our device fabrication techniques can selectively choose a SWNT diameter for the platform, and it can be used to explore the unique trend near 1.6 nm range. Two devices fabricated to have multiple-SWNT channels show similar enhancement with each containing one SWNT in the vicinity of 1.6 nm (1.57 and 1.58 nm), further supporting the trend. Using the observed maximum, it was possible to assign blocking events to specific individual SWNTs. For example, a device with two SWNTs of diameter 1.6 and 1.8 nm that exhibited two sets of stochastic behaviour with very different pore-blocking currents, could be assigned with the knowledge that there is a strong peak in pore-blocking current at 1.6 nm. We used this data to supplement the trends in the single-device data. The assignment of metallic or semiconducting of each SWNT was determined from Raman characterization, but somewhat surprisingly, the designation does not seem to correlate with observed transport characteristics. All data points from each device are shown as scatter plots (see Supplementary Figs S5–S7 ). 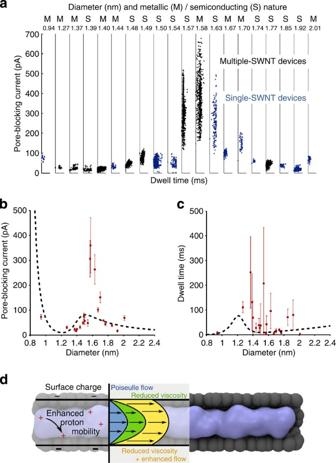Figure 5: Diameter dependence of ion transport phenomena. (a) Pore-blocking current for each device separated by observed dwell time, with diameter and metallic/semiconductor nature marked.xAxis is displayed on a log scale (100–103(ms)), all tested with 3 M KCl and 1 V applied voltage. (b,c) Observed pore-blocking current and dwell time as a function of SWNT diameter, along with the results from the electrochemical model. Error bars represent the range of measurements over the many stochastic events for each SWNT. (d) Illustration of the physical effects accounted for in the electrochemical model. Figure 5: Diameter dependence of ion transport phenomena. ( a ) Pore-blocking current for each device separated by observed dwell time, with diameter and metallic/semiconductor nature marked. x Axis is displayed on a log scale (10 0 –10 3 (ms)), all tested with 3 M KCl and 1 V applied voltage. ( b , c ) Observed pore-blocking current and dwell time as a function of SWNT diameter, along with the results from the electrochemical model. Error bars represent the range of measurements over the many stochastic events for each SWNT. ( d ) Illustration of the physical effects accounted for in the electrochemical model. Full size image Temperature dependence of transport phenomena The temperature dependence of pore blocking can shed light on the transport mechanism, and determine the influence of structured, solid water as suggested in simulations [27] , [37] . Reversibly heating the platform ( Fig. 6a ) to 50 °C while recording I BC was used to explore three single SWNT devices of unassigned diameter (see the Methods and Supplementary Note 5 ). Room temperature I BC data suggest that one SWNT (red) lies near 1.6 nm and the other two do not. I BC decreases with an Arrhenius dependence ( Fig. 6b ) for all three with apparent activation energies of 6, 11, 15 kcal mol −1 (see Supplementary Table S2 ). These values are larger than the activation energies necessary for accelerated proton transport via the Grotthus mechanism alone, which is estimated at only 2–3 kcal mol −1 (refs 9 , 38 ). Possible sources of this activation energy are the presence of an energy barrier at the SWNT entrance or exit region, or a secondary effect from temperature dependence of the proton-water equilibrium [39] . Especially, the energy barrier near the entrance might be due to the desolvation of a cation species in going into one SWNT [40] , with an activation energy of about 12 kcal mol −1 activation [41] . Also, transition of atomic water density structures depending on temperature changes [37] might affect the requirement of energy to occupy the nanoscale channels by the blockers. Most interesting is that there is not a discontinuity indicative of a phase transition, suggesting that a liquid water phase is present throughout our diameter range. Similar temperature scaling data are shown in Fig. 5d for the dwell time, with the SWNT near 1.6 nm (red) decreasing as temperature increases. The trend for SWNT3 is opposite. Such diverse behaviour is perhaps anticipated by the non-monotonic trends with diameter uncovered in this work, motivating further study of SWNT transport in this range. 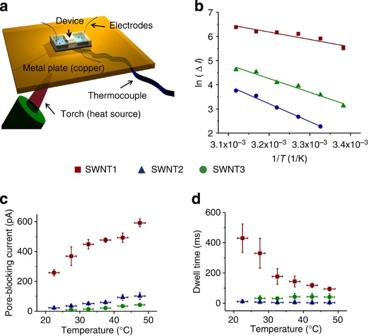Figure 6: Temperature dependence of ion transport for three single-SWNT devices. (a) Illustration of the modified setup for temperature-dependent measurements. (b) Arrhenius plot of the pore-blocking current for the three devices. (c,d) Pore-blocking current and dwell time for each device over the range of tested temperatures. Error bars represent the range of transport measurements for each SWNT at each temperature. Figure 6: Temperature dependence of ion transport for three single-SWNT devices. ( a ) Illustration of the modified setup for temperature-dependent measurements. ( b ) Arrhenius plot of the pore-blocking current for the three devices. ( c , d ) Pore-blocking current and dwell time for each device over the range of tested temperatures. Error bars represent the range of transport measurements for each SWNT at each temperature. Full size image Our results are easily understood within a simple electrochemical model building upon previous theoretical studies on the diameter dependence of transport through SWNTs. Water confined in nanopores of diameter similar to its molecular size demonstrates slip-flow at the walls [31] , reduced viscosity [42] and increased proton transport rates [23] . Both protons and blocking ions within a SWNT will feel these effects and our simple model, illustrated in Fig. 5d , builds upon these studies to reproduce the transport maximum that we observe experimentally. We note that previous transport models proposed to explain similar effects [21] do not explicitly contain the diameter dependencies in all parameters. First, we assume a fitted diameter-independent linear charge density on the SWNT, similar to that of previous works [21] , that results in a net positive proton concentration in the SWNT interior. With the much larger aspect ratio, we expect a more linear electric field throughout most of the length of our device than previous studies [21] , resulting in convective proton transport as well as diffusive proton transport if the SWNT is not blocked with a larger cation. If the protons are unable to interact directly with the SWNT walls, the energy being dissipated at steady state from the electric field must be dissipated to the surrounding fluid in the SWNT. We model this proton driving force as an effective pressure that drives water convection. At steady state, the energy required for hydrodynamic flow (lhs) is balanced by the energy of proton transport through the electric field (rhs), hence: for the open channel state and for the blocked state. Here and are the mean fluid velocity in the SWNT in the open and blocked states, respectively, η is a diameter-dependent water viscosity [42] , D is the SWNT diameter, are the proton concentration (balancing the SWNT charge) in the open and blocked states, respectively, μ H ( D ) is the diameter-dependent proton mobility, E f is the uniform electric field magnitude and ε is a diameter-dependent enhancement factor fitted to smoothly represent literature simulation results [31] that represents deviations in fluid transport from an ideal Poiseuille flow through a pipe of equivalent diameter (see Supplementary Note 4 and Supplementary Fig. S12 ). We approximate the proton mobility with an exponential interpolation between the small diameter-enhanced rate mobility [23] and bulk transport rates [43] . We note that most of the properties are strongly diameter dependent, currently not well-understood, and with varying values in literature, as only simulation results have been available to date without an experimental platform for validation. The proton concentration is assumed to be diameter independent and influenced by whether the SWNT is blocked by a translocating ion. After solving for the open and blocked fluid velocities, and , the key experimentally observable quantities can be calculated: and, assuming the ion is carried in the convective flow, the dwell time τ = L / , where L is the length of the SWNT. Although our model uses two fitted parameters as in previous literature studies [21] , the SWNT surface charge in the open and closed state, , affect only the magnitude of the pore-blocking current and dwell time and not the characteristic diameter dependence we report here. A comparison of our experimentally determined diameter dependence and this electrochemical model are shown in Fig. 5b,c . Critically, we note that the position of the local maximum in Fig. 5b is approximately reproduced at 1.5 nm compared with 1.6 nm observed, primarily through the strong diameter dependence of ε . There is an increasing trend of I BC as diameter decreases for D <1.2 nm as the water structure becomes more important and at large diameters ( D >1.9 nm) as transport approaches the bulk (Poiseuille) case. The overall trend of I BC is similar as it is fitted through the proton concentrations, but the model predicts a smaller peak in the blockade current at the 1.6 nm local maximum found experimentally. There is less agreement between this model and the observed dwell times, but the predicted times are within an order of magnitude. Also, there is a hypothesis about the change of coordination number of ions near this critical diameter. It is well known that the bulk hydration radius is not the same as that in the nano-confined structures. However, it is not known which channel sizes tend to shed hydration shells and change hydrated radius to accept the specific ions. Changing the cation type could alter the precise location of this transition region based on the ion hydration structure, but this is unexplored in this work aside from noting the ionic dependence on the blockade current and dwell time. In conclusion, the first experimental support for non-monotonic diameter-dependent transport in SWNTs is demonstrated and analysed. We expect further simulation and theoretical study to elucidate the precise mechanisms behind these effects. These results highlight several outstanding issues that prevent the prediction of these phenomena from first principles. An obvious extension to a quantitative understanding of these effects would be the design of functionalized SWNT with specific diameters to optimally transport or filter new molecules of interest. Growth of ultra-long aligned SWNTs The platform is constructed using an epoxy structure that acts as both an oxygen plasma mask for the opening of the nanotube ends and to form two liquid reservoirs at either side. The SWNTs are synthesized and aligned using by methane CVD in a horizontal quartz tube furnace with an inner diameter of 22 mm (CVD furnace: Thermo Fisher Scientific Lindberg/Blue M * 1,100 °C, TF55035A, Mass flow controller: Aalborg SDPROC Microprocessor Driven Command Module). After a catalyst layer, 0.5-nm-thick Fe was deposited on a Si/SiO 2 wafer by electron beam evaporation, the substrate was placed in the quartz tube. Methane (CH 4 ) was used as the carbon source. Hydrogen (H 2 ) and argon (Ar) were used as catalysts and carrier gases, respectively. The flow rate was 3 sccm of H 2 during increase of temperature up to 950 °C for 46 min, and the temperature and the flow rate were maintained for 30 min. Next, the temperature was increased up to 1,015 °C for 33 min. After these steps, CH 4 was introduced into the furnace at 1,015 °C and 1 atm, and ultra-long aligned SWNTs were grown for 3 h 30 min. Characterization of a single SWNT by Raman spectroscopy The diameter and metallicity of each carbon nanotube used in devices for the diameter study was characterized using Raman spectroscopy (Horiba LabRAM HR). In order to locate individual SWNTs, optically observable markers were placed on the substrate and imaged in a scanning electron microscope, which can be used to image carbon nanotubes. The relative distance between the marker and SWNT were used to locate the SWNT in the Raman’s optical microscope. A 633-nm laser excitation source was predominantly used to identify the SWNT, although a 532-nm laser excitation source was also used in some cases. From the Raman spectrum, the RBM peak position has been found to be inversely related to the carbon nanotube diameter through the following relation: d t =248/ ω RBM , which is valid for isolated SWNT sitting on a silicon oxide substrate [34] . The Raman RBM spectra for all 20 different nanotube diameters are shown in Supplementary Fig. S2 . One device actually contained a double-walled carbon nanotube as indicated by the presence of two RBM peaks; in this case, the smaller, inner tube’s diameter was used. The G band of the carbon nanotube corresponds to tangential vibrations of the carbon atoms in the carbon nanotube, and it is observed at higher wavenumber shifts (~ 1,550–1,600 cm −1 ) in the Raman spectrum. The G band contains two peaks, the G − and G + peaks, where the G + peak stays mostly constant around 1,591 cm −1 and the G − peak is at lower wavenumber shifts and changes more dramatically. The shape of the G − peak gives evidence of the metallicity of the tube. Metallic tubes have broader G − peaks that are softened compared with those of semiconducting tubes. Metallic G − peaks can also be fitted to a Breit-Wigner-Fano lineshape, compared with a Lorentzian lineshape for those of semiconducting tubes [44] . The deconvoluted Raman G band spectra for all 20 different nanotube diameters are shown in Supplementary Fig. S2 , with the G − peak fitted to a Breit-Wigner-Fano or Lorentzian (depending on whether the nanotube was determined to be metallic or semiconducting), and the G + peak fitted to a Lorentzian. In several cases, an additional peak was observed, which was thought to be due to amorphous carbon around the SWNT from the growth process. The criteria used to determine the metallicity of the tube was by first looking for distinctly broad or sharp G − peaks, which would indicate that the nanotube was metallic or semiconducting, respectively. For tubes whose assignment was still ambiguous, the position of the G − peak was used to determine the metallicity, as metallic tubes have softened G − phonon modes relative to semiconducting tubes. The empirical fits from Jorio et al. 44 were used to assign metallicity to the ambiguous tubes, as shown in Supplementary Fig. S3 . The diameters and metallicity of all the nanotubes are summarized in Supplementary Table S1 . Device fabrication and measurement of the pore blocking Horizontally aligned SWNT were grown using CVD. The specific markers that indicate the position of SWNTs on silicon wafer were deposited by E-beam evaporation technique. At this stage, SWNTs on the specific area were characterized by Raman spectra, which would give the information of diameters and types (metal or semiconducting) of SWNTs. According to the collected information, the only one SWNT was chosen and remained as the specific nanochannel in the device, whereas all other SWNTs were removed by a razor blade etching process. SU-8 photoresist was used to fabricate the epoxy structure for reservoirs of ionic solution and a mask against plasma etching. A constant-volume-injection method with spin coating was used to construct an ultra-thick SU-8 epoxy structure. The epoxy structure was glued onto the silicon wafer containing one ultra-long aligned SWNT using a ultraviolet-curing optical adhesive (Norland) to form a tight seal. The plasma etch removes an exposed SWNT leaving 1 mm across the protected section, and opens both ends at the bottom of epoxy reservoirs. The duration of oxygen plasma etching was optimized to remove the exposed parts of a SWNT and not to etch out the nanofluidic part of a SWNT underneath the epoxy wall. Scanning electron microscope images were recorded during the process, repeatedly. With both compartments filled with approximately 15–60 μl aqueous ionic solution (KCl, LiCl, NaCl, CsCl, CaCl 2 ), ion current across the reservoirs was monitored using Axopatch 200B (Molecular Devices, 2 kHz Bessel low-pass filter, 250 kHz acquisition frequency). Ag/AgCl electrodes are used to apply electric field across the reservoirs. Successful device manufacturing rate A number of devices with one, two or three SWNTs were fabricated and tested for ion translocation with a voltage clamp setup. A higher failure rate has been observed in a device with a single SWNT compared with multi-SWNT devices. In the previous work, multiple SWNTs in one device were fabricated to increase the probability of the observation of ion transport during experiments. Many SWNTs in multi-SWNT devices were permanently blocked by impurities or defects from CVD or fabrication processes. Moreover, SWNTs with a high aspect ratio might be bent or damaged during the fabrication, and these uncertain obstructions could block the paths of ions. An applied electric field (maximum 1,000 mV) may also be below the necessary field to begin ion translocation by cleaning the blocking species or to overcome the potential barrier (threshold voltage) near the pore mouth. Therefore, many devices were fabricated and tested. Pore-blocking events were identified in about 15 devices out of over 100 devices. Temperature dependence experiments In order to determine the effect of temperature on observed transport characteristics, the devices were heated during a typical voltage clamp experiment. Because of the low currents being measured (picoamps), a butane torch was used as the heating device, as opposed to a hot plate, which produced too much interfering electrical noise. Supplementary Fig. S13 is a photo of the temperature scaling setup. The torch is fixed to the optical table and directed towards the sample, which is placed on a thermally conductive surface. A thermocouple placed close to the sample is used to record the temperature in real time. During the experiment, the torch was turned on when regular pore blocking events are observed, using the same 3 M KCl solution as in the diameter experiments. Supplementary Fig. S14 shows the typical temperature response from application of the torch. The temperature during this experiment was kept under 50 °C to avoid excessive evaporation. According to the calibration process, we found that applying heat from the torch for 7 s would increase the temperature up to 50 °C. Because of the heat transfer delay, the temperature reaches the maximum after 20 s of stopping the torch. After the maximum temperature is reached, the system cools down slowly through heat transfer to the environment. During this time, ion transport events are monitored using the voltage clamp apparatus and correlated to specific temperatures. How to cite this article: Choi, W. et al. Diameter dependent ion transport through the interior of isolated single walled carbon nanotubes. Nat. Commun. 4:2397 doi: 10.1038/ncomms3397 (2013).